Copper-catalyzed remote C(sp3)–H azidation and oxidative trifluoromethylation of benzohydrazides 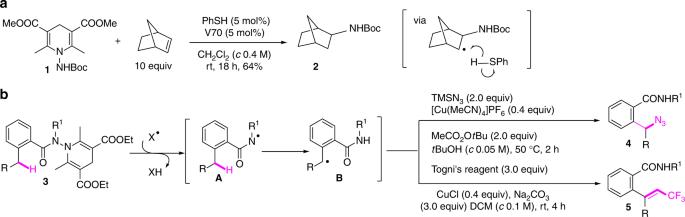Fig. 1 Amidyl radicals and HLF reaction.aStuder’s work on the use ofN-aminated dihydropyridines as precursors ofN-centered radicals: hydroamination of alkenes;bbenzohydrazides in HLF reaction: functionalization of remote C(sp3)–H bond. V70 = 2,2’-azobis(2,4-dimethyl-4-methoxy valeronitrile); TMSN3= trimethylsilyl azide; MeCO2OtBu =tert-butyl peroxyacetate The Hofmann-Löffler-Freytag (HLF) reaction is a prototypical example of radical-based remote functionalization of unactivated C( sp 3 )–H bond. While 1,5-hydrogen atom transfer (1,5-HAT) of the amidyl radical is thermodynamically favorable and is well-established, the method for the subsequent functionalization of the translocated carbon radical is still limited. We report herein two catalytic remote C( sp 3 )–H functionalization protocols. Cu(MeCN) 4 PF 6 -catalyzed reaction of 2-alkyl benzohydrazides 3 with TMSN 3 in the presence of MeCO 2 O t Bu affords the γ-azido amides 4 , while CuCl-catalyzed reaction of 3 with Togni’s reagent provides 2-(β-trifluoromethylvinyl)benzamides 5 via an oxidative δ-trifluoromethylation of the alkyl group. 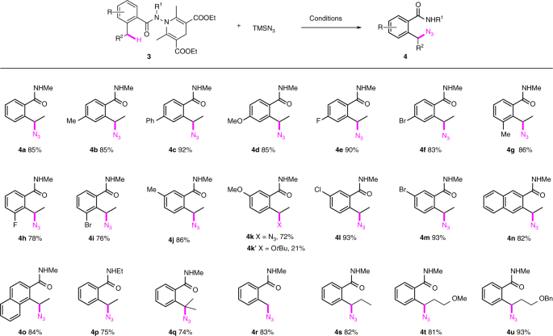Fig. 2 γ-Azidation of 2-alkyl benzohydrazides.3(0.1 mmol), TMSN3(0.2 mmol), Cu(MeCN)4PF6(0.04 mmol), MeCO2OtBu (0.2 mmol),tBuOH (2.0 mL,c0.05 M), 50 °C, 2 h Mechanistic studies suggest that the γ-azidation of benzohydrazides 3 goes through 1,5-HAT followed by a Cu-mediated azido transfer cascade, while the oxidative δ-trifluoromethylation of 3 proceeds via, after 1,5-HAT process, a radical-polar crossover mechanism. The Hofmann–Löffler–Freytag (HLF) reaction [1] , [2] that converts the N -haloamines to pyrrolidines constitutes a prototypical example of radical-based remote C( sp 3 )–H bond functionalization process [3] . The reaction, discovered in 1883, is a complex domino process involving the generation of the aminium radical followed by regioselective 1,5-hydrogen atom transfer (HAT), halogenation, and cyclization [4] , [5] , [6] , [7] , [8] . The instability of the N -haloamines, as well as the generally harsh conditions required for the generation and subsequent hydrogen atom abstraction of aminium radicals, limited nevertheless the full exploitation of its synthetic potential. A major breakthrough addressing this issue came from Suárez’s group. In a series of seminal papers, they reported that amides/sulfonamides can be converted to the corresponding amidyl and sulfonamidyl radicals with iodine/lead tetraacetate [9] , [10] or iodine/phenyliodine diacetate [11] as oxidants, and these electron-withdrawing group-attached nitrogen-centered radicals readily undergo intramolecular HAT under mild neutral conditions. Recently, Müniz et al. [12] , [13] , [14] , [15] showed that the amidyl radical can be generated directly from the secondary amide under mild catalytic oxidative conditions, while the group of Knowles [16] and Rovis [17] , [18] demonstrated independently that photoredox conditions were very effective for the same purpose. Complementary to this work, significant efforts have also been made recently in identifying tailored precursors for the generation of the N -centered radicals [19] , [20] , [21] , [22] , [23] , [24] , [25] . The development of these easily available and stable amidyl radical precursors in conjunction with the recent advent of metal and visible-light photoredox catalysts allowed the execution of the HLF reaction under much milder conditions, therefore providing opportunities to expand the repertoire of the remote C( sp 3 )–H functionalization process. Indeed, besides the cyclization to N -heterocycles [9] , [10] , [11] , [26] , [27] , [28] , [29] , [30] , [31] , [32] , halogenation [22] , [23] , [33] , [34] , [35] , [36] and C–S bond formation [21] that are inherent to the classic radical chain mechanism of the HLF reaction, C–C bond formation via radical addition [16] , [17] , [18] , [37] , [38] , [39] , azidation/cyanation [19] , [20] , [22] , acetoxylation [40] , thiolation/alkynylation [20] , [22] , and arylation [24] , [25] have been developed very recently. Studer et al. demonstrated that amidyl radicals can be generated from N -aminated dihydropyridines 1 and be used in the hydroamination of olefins (Fig. 1a ) [41] , [42] . Mechanistically, the process is initiated by the polarity-matched abstraction of the Hantzsch ester’s C-4 hydrogen by the electrophilic thiophenol radical to afford, after fragmentation, the amidyl radical and pyridine. The addition of the former to the double bond followed by hydrogen transfer from thiophenol to the resulting radical adduct afforded the product 2 with concurrent regeneration of the thiophenol radical to propagate the chain. Inspired by these results and in connection with our interest in remote C( sp 3 )–H functionalization processes [24] , [43] , [44] , we hypothesized that if the amidyl radical A was generated by action of an electrophilic radical species (X•) whose reduced form X–H was reluctant to transfer its hydrogen to the relayed C -centered radical B , then it would be possible to functionalize B by other reactive species to afford remote functionalized amides. We assumed that electrophilic trifluoromethyl and tert -butoxy radicals could satisfy these criteria as CF 3 –H and t BuO–H would not be able to propagate the chain reaction due to their high bond dissociation energies (CF 3 –H: 107.4 kcal/mol, t BuO–H: 106.3 kcal/mol). We report herein the Cu-catalyzed γ-azidation and oxidative δ-trifluoromethylation of benzohydrazides 3 for the synthesis of amides 4 and 5 , respectively (Fig. 1b ). Conversion of ethyl to trifluoromethylvinyl group is, to the best of our knowledge, unknown. Fig. 1 Amidyl radicals and HLF reaction. a Studer’s work on the use of N -aminated dihydropyridines as precursors of N -centered radicals: hydroamination of alkenes; b benzohydrazides in HLF reaction: functionalization of remote C( sp 3 )–H bond. V70 = 2,2’-azobis(2,4-dimethyl-4-methoxy valeronitrile); TMSN 3 = trimethylsilyl azide; MeCO 2 O t Bu = tert -butyl peroxyacetate Full size image Cu-catalyzed γ-C( sp 3 )–H azidation of benzohydrazides While azidation of alkenes are well developed [45] , [46] , [47] , [48] , direct azidation of C( sp 3 )–H bond remains challenging [49] . Indeed, the γ-azidation of amides was unknown at the outset of this work. However, Studer et al. have very recently reported such a transformation using TfN 3 as an azide donor [19] . We focused on the use of stable and readily available TMSN 3 as an azide source and the benzohydrazides 3 [41] , [42] as precursors of amidyl radicals. In line with our working hypothesis and knowing that peroxide is compatible with the Cu-catalyzed carboazidation process [50] , [51] , the reaction of 3a (R 2 = Me, R = R 1 = H) with TMSN 3 was investigated in the presence of copper salts and peroxides. After systematic screening of the copper sources [CuCl, CuBr, CuI, CuOTf·benzene, Cu(MeCN) 4 PF 6 , Cu(OAc) 2 , Cu(OTf) 2 , CuSO 4 , Cu(acac) 2 , Cu(ClO 4 ) 2 ], the peroxides ( t BuOOH, t BuOO t Bu, cumene hydroperoxide, PhCO 2 O t Bu, MeCO 2 O t Bu), and the solvents ( t BuOH, DCE, 1,4-dioxane, MeCN, CF 3 CH 2 OH), the optimum conditions found consisted of heating a t BuOH solution of 3a ( c 0.05 M) and TMSN 3 (2.0 equiv) at 50 °C in the presence of Cu(MeCN) 4 PF 6 (0.4 equiv) and MeCO 2 O t Bu (2.0 equiv, 50 wt. % in odorless mineral spirits from Sigma). Under these conditions, the azido amide 4a was isolated in 85% yield (Fig. 2 ). A small amount of 2-(1-( tert -butoxy)ethyl)- N -methylbenzamide (see Supplementary Information) was also isolated from the reaction mixture. Fig. 2 γ-Azidation of 2-alkyl benzohydrazides. 3 (0.1 mmol), TMSN 3 (0.2 mmol), Cu(MeCN) 4 PF 6 (0.04 mmol), MeCO 2 O t Bu (0.2 mmol), t BuOH (2.0 mL, c 0.05 M), 50 °C, 2 h Full size image The scope of this azidation protocol was next examined (Fig. 2 ). A range of 2-alkyl substituted benzohydrazides were converted to the corresponding 2-(1-azidoalkyl)benzamides in good-to-excellent yields. Halides (F, Cl, Br) at different position of the aromatic ring was compatible with the reaction conditions affording the azido derivatives suitable for further functionalization. The primary, secondary, and tertiary benzylic carbons were all successfully functionalized to afford the corresponding azides in good to excellent yields. In the case of 3k (R = 4-MeO), the desired azido compound 4k (72%) was isolated together with a significant amount of 4k’ (X = O t Bu, 21%) probably due to the presence of a strong electron-donating para -methoxy group. A series of control experiments were carried out to gain insight on the reaction mechanism. Treatment of N -methyl-2-ethylbenzamide ( 6 ) under standard conditions failed to produce even a trace amount of azido amide 4a indicating that 6 was not an intermediate of the reaction (Fig. 3 , a ). In line with the radical mechanism, azidation of 3a was completely inhibited in the presence of TEMPO or BHT, and a radical clock experiment involving cyclopropane-containing substrate 7 afforded azide 8 in 65% yield (Fig. 3 , b ). 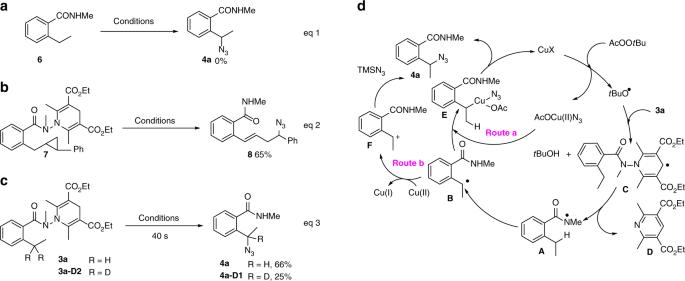Fig. 3 Mechanistic studies on the γ-azidation of 2-alkyl benzohydrazides.aControl experiment;bradical clock experiment;cKIE experiment;dpossible reaction pathway; conditions:6,7or3a/3a-D2(0.1 mmol), TMSN3(0.2 mmol), Cu(MeCN)4PF6(0.04 mmol), MeCO2OtBu (0.2 mmol),tBuOH (2.0 mL,c0.05 M), 50 °C, 2 h A side-by-side kinetic experiment using 3a and 3a-D2 provided an intermolecular KIE value of 2.6 (Fig. 3 , c ) suggesting that the 1,5-HAT, an off-catalytic cycle process, might be a rate-limiting step in the present domino azidation process. Fig. 3 Mechanistic studies on the γ-azidation of 2-alkyl benzohydrazides. a Control experiment; b radical clock experiment; c KIE experiment; d possible reaction pathway; conditions: 6 , 7 or 3a/3a-D2 (0.1 mmol), TMSN 3 (0.2 mmol), Cu(MeCN) 4 PF 6 (0.04 mmol), MeCO 2 O t Bu (0.2 mmol), t BuOH (2.0 mL, c 0.05 M), 50 °C, 2 h Full size image On the basis of these results, a possible reaction pathway for the γ-azidation of benzohydrazide 3a is proposed (Fig. 3 , d ). Reduction of peroxide by Cu(I)X salt would produce AcOCuX salt and tert -butoxy radical, which would abstract the C-4 hydrogen from dihydropyridine to give t BuOH and dihydropyridine radical C . Fragmentation of the latter would lead to the amidyl radical A and pyridine D . Subsequent 1,5-HAT of A would generate the benzyl radical B which, upon radical rebound with AcOCu(II)N 3 (Fig. 3 , d , route a), would afford Cu(III) species E . Reductive elimination would then deliver the γ-azido amide 4a with the concurrent release of Cu(I) salt. The formation of 2-(1-( tert -butoxy)ethyl)- N -methylbenzamide could be accounted for by the presence of minor amount of t BuOCuX species in the reaction mixture [52] . An alternative pathway would involve the oxidation of radical B to benzyl cation F that could then be trapped by TMSN 3 to provide 4a (Fig. 3 , d , route b). To verify this possibility, the reaction of 3o (R = 5-OMe, cf Fig. 2 ) with TMSN 3 was carried out in a mixture of solvent ( t BuOH/MeOH = 1:1) under otherwise identical conditions. Azide 4o was still isolated in 65% yield together with a small amount of 2-(1-( tert -butoxy)ethyl)- N -methylbenzamide (6%). Methoxylated product was not observed. This result together with the fact that isoindolinone [53] , [54] , [55] was not formed under our conditions are in accord with the Cu-mediated redox azido transfer mechanism [50] , [51] . Cu-catalyzed oxidative δ-C( sp 3 )-trifluoromethylation Trifluoromethylation of 2-alkyl benzohydrazides was next examined. The reaction of 3a with Togni’s reagent 9 [46] , [47] , [48] in the presence of metal salts was chosen as a benchmark reaction. Instead of obtaining the N -methyl-2-(1,1,1-trifluoropropan-2-yl)benzamide, our initial experiments allowed us to isolate unexpectedly the compound 5a whose structure was confirmed by X-ray crystallographic analysis (Fig. 4 ). Since the reaction converting formally an ethyl group to a trifluoromethylvinyl group was unknown [56] , conditions were further optimized toward its formation by varying the catalysts (Cu(I), Cu(II), Fe(II), Fe(III) salts), the solvents (DCM, DCE, toluene, 1,4-dioxane), and the additives (NaHCO 3 , Na 2 CO 3 , K 2 CO 3 , NaH 2 PO 4 , etc.) (see Supplementary Information). The optimum conditions found consisted of stirring a solution of 3a and Togni’s reagent 9 (3.0 equiv.) in DCM ( c 0.10 M) in the presence of CuCl (0.4 equiv.) and Na 2 CO 3 (3.0 equiv.) at room temperature. Under these conditions, 5a was isolated in 74% yield. Fig. 4 Oxidative δ-trifluoromethylation of 2-alkyl benzohydrazides. 3 (0.1 mmol), Togni’s reagent 9 (0.3 mmol), CuCl (0.04 mmol), DCM (1.0 mL), Na 2 CO 3 (0.3 mmol), rt, 4 h Full size image The generality of this oxidative γ-trifluoromethylation of 2-ethyl benzohydrazides was next examined (Fig. 4 ). The presence of the electron-donating (Me, OMe) and -withdrawing groups (CN) and halides (F, Cl, Br, I) at different positions of the aromatic ring were well tolerated to afford the corresponding 2-(β-trifluoromethylvinyl)benzamides (5a–5q) in good yields. In the case of 3 m (R = 3-Br), the corresponding isoindolinone resulting from the intramolecular C–N bond formation was isolated in 5% yield. N -methyl 3-ethyl and N -methyl 1-ethyl-2-naphthohydrazides were similarly transformed to the corresponding β-trifluoromethylvinyl substituted naphthoamides 5r and 5 s . The N ,2-diethyl benzohydrazide was chemoselectively converted to N -ethyl-2-(β-trifluoromethylvinyl)benzamide 5t without event. Finally, 2-isopropyl benzohydrazide was converted to a mixture of two isomers 5 u / 5 u’ (1:1) in a moderate yield. The methyl amide 5a was readily hydrolyzed to the corresponding carboxylic acid 5 v (HOAc–H 2 O, 20% H 2 SO 4 ), providing therefore a versatile functional group for further functionalization. Addition of TEMPO to the reaction of 3a with 9 inhibited completely the process and only 2,2,6,6-tetramethyl-1-(trifluoromethoxy)piperidine was formed. Reducing the amount of Togni’s reagent 9 to 1.5 equiv. under otherwise identical conditions decreased the yield of 5a (42% yield) with concurrent formation of N -methyl-2-vinyl benzamide ( 10 ) and N -methyl-2-ethylbenzamide ( 6 ) in yields of 12 and 4%, respectively (Fig. 5 , a ). Resubmitting 10 to the standard conditions afforded 5a in 89% yield [57] , while 6 remained unchanged under standard conditions. A side-by-side experiment using 3a and 3a-D2 provided an intermolecular KIE (k H /k D ) value of 2.3 indicating that the 1,5-HAT step could be a rate-limiting step in our domino process (Fig. 5 , b ). Finally, treatment of 3r under standard conditions furnished 11 in 36% yield. This result indicated that the 1,5-HAT of the in situ generated amidyl radical occurred. However, in contrast to the azidation process, the transfer of CF 3 to the resulting translocated benzyl radical was not fast enough to compete with the intramolecular C–N bond formation (Fig. 5 , c ). Fig. 5 Mechanistic studies on the oxidative δ-trifluoromethylation of 2-alkyl benzohydrazides. a Control experiment; b KIE experiment; c isoindolinone formation; d possible reaction pathway; conditions: 10 or 6 or 3a/3a-D2 (0.1 mmol), Togni’s reagent 9 (0.3 mmol), CuCl (0.04 mmol), DCM (1.0 mL, c 0.1 M), Na 2 CO 3 (0.3 mmol), rt, 4 h Full size image On the basis of the results of these control experiments, a possible reaction pathway is proposed (Fig. 5 , d ). Single-electron transfer between Togni’s reagent 9 and CuCl would produce the CF 3 radical and Cu(II) salt G . The abstraction of the C-4 hydrogen of the Hantzsch ester 3a by CF 3 • generated radical C which underwent fragmentation to provide the amidyl radical A and pyridine D . The 1,5-HAT of A furnished the then translocated benzyl radical B , which upon radical rebound with Cu(II) salt G , would afford H . 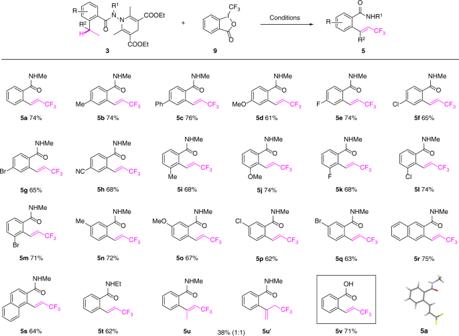Fig. 4 Oxidative δ-trifluoromethylation of 2-alkyl benzohydrazides.3(0.1 mmol), Togni’s reagent9(0.3 mmol), CuCl (0.04 mmol), DCM (1.0 mL), Na2CO3(0.3 mmol), rt, 4 h Reductive elimination leading to the formation of C–Cl and C–OCOAr bonds may not be kinetic competent, the alternative β-hydride elimination took place to afford 2-vinyl benzamide ( 10 ). Subsequent addition of CF 3 radical to the newly generated double bond would generate the benzyl radical I which, upon radical rebound and β-hydride elimination, would afford the observed product 5a with concurrent generation of the Cu(I) species. Following this reaction pathway, at least two equivalents of Togni’s reagent 9 are needed to complete this domino process, which is in accordance with the result of our control experiment. Post-transformations of azido amide 4a were carried out to illustrate its synthetic potential (Fig. 6 ). Chemoselective reduction of the amide function in 4a with Schwartz’s reagent delivered azido aldehyde 12 in 76% yield. Heating to reflux a MeOH solution of 4a with indium in the presence of NH 4 Cl afforded the isoindolinone 13 in 91% yield via probably a reduction/transamidation sequence. 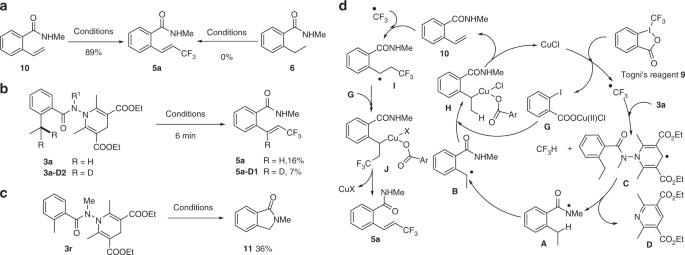Fig. 5 Mechanistic studies on the oxidative δ-trifluoromethylation of 2-alkyl benzohydrazides.aControl experiment;bKIE experiment;cisoindolinone formation;dpossible reaction pathway; conditions:10or6or3a/3a-D2(0.1 mmol), Togni’s reagent9(0.3 mmol), CuCl (0.04 mmol), DCM (1.0 mL,c0.1 M), Na2CO3(0.3 mmol), rt, 4 h 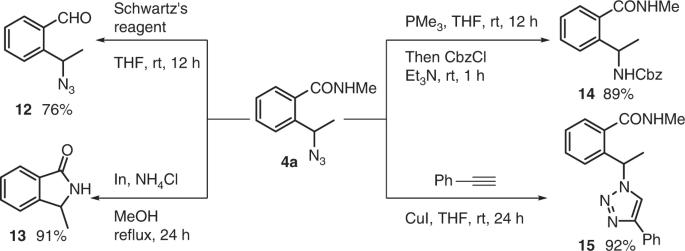Fig. 6 Transformation of azido amide4a. Schwartz’s reagent = bis(cyclopentadienyl)zirconium(IV) chloride hydride, CbzCl = benzyl chloroformate On the other hand, Staudinger reduction of azide followed by in situ acylation with CbzCl furnished carbamate 14 , while the click reaction of 4a with phenylacetylene provided the triazole 15 in 92% yield. Fig. 6 Transformation of azido amide 4a . Schwartz’s reagent = bis(cyclopentadienyl)zirconium(IV) chloride hydride, CbzCl = benzyl chloroformate Full size image The classic Hofmann–Löffler–Freytag (HLF) reaction converts the protonated N -chloroamines to pyrrolidines under thermal or photochemical conditions. In this transformation, the carbon-centered radical, resulting from the 1,5-HAT of the in situ generated aminium radical, abstracts a chlorine atom from the ammonium salt forming therefore a radical chain process. While many different transformations could in principle be envisaged for the functionalization of the translocated C-centered radical, only very few reaction types have actually been successfully combined with the 1,5-HAT process. In this paper, we presented two copper-catalyzed remote C( sp 3 )–H functionalization processes in which the metal-catalyzed cross-coupling reactions were successfully merged with the radical 1,5-HAT process. The salient feature of these transformations was that the copper salts served not only as a reductant to generate the amidyl radicals from benzohydrazides 3 , but also catalyzed the functionalization of the translocated carbon radical. Specifically, Cu(MeCN) 4 PF 6 -catalyzed reaction of 2-alkyl benzohydrazides 3 with TMSN 3 in the presence of MeCO 2 O t Bu affords the γ-azido amides 4 , while CuCl-catalyzed reaction of 3 with Togni’s reagent provides 2-(β-trifluoromethylvinyl)benzamides 5 via an oxidative δ-trifluoromethylation of the alkyl group. Mechanistic studies suggest that the γ-azidation of benzohydrazides 3 goes through 1,5-HAT followed by a Cu-mediated azido transfer cascade, while the oxidative δ-trifluoromethylation of 3 proceeds via, after 1,5-HAT process, a radical-polar crossover mechanism. In view of the availability and reliability of a wide range of metal-catalyzed cross-coupling reactions, we believe that their combination with the 1,5-HAT process will open a new avenue for the development of powerful synthetic tools [58] . Cu-catalyzed γ-C( sp 3 )–H azidation of benzohydrazides A screw cap tube was charged with Cu(CH 3 CN) 4 PF 6 (14.9 mg, 0.04 mmol, 0.4 equiv. ), substrate 3 (0.1 mmol, 1.0 equiv. ), TMSN 3 (26.5 μL, 0.2 mmol, 2.0 equiv. ), and t BuOH (2.0 mL). The mixture was stirred at 50 °C for 2 min, then MeCO 2 O t Bu (32.2 μL, 0.2 mmol, 2.0 equiv.) was added to the above mixture. After being stirred for 2 h at 50 °C under N 2 atmosphere, the reaction mixture was quenched with water, extracted with EtOAc. The organic extracts were washed with brine, dried over Na 2 SO 4 . The solvent was removed under reduced pressure. The residue was purified by flash column chromatography (SiO 2 , eluent: petroleum ether/EtOAc = 2/1) to give 4 . Cu-catalyzed oxidative δ-C( sp 3 )–H trifluoromethylation To a screw cap tube charged with CuCl (4.0 mg, 0.04 mmol, 0.4 equiv.) and Na 2 CO 3 (31.8 mg, 0.3 mmol, 3.0 equiv.) was added a solution of Togni’s reagent 9 (94.8 mg, 0.3 mmol, 3.0 equiv.) in DCM (0.5 mL) under argon atmosphere. After stirring for 2 min, substrate 3 (0.1 mmol, 1.0 equiv.) in DCM (0.5 mL) was added to the above mixture. After being stirred for 4 h at room temperature under argon atmosphere, the reaction mixture was quenched with water, extracted with EtOAc. The organic extracts were washed with Na 2 CO 3 solution and brine, dried over Na 2 SO 4 . The solvent was removed under reduced pressure. The residue was purified by flash column chromatography (SiO 2 , eluent: petroleum ether/EtOAc = 2/1) to give 5 .